Quantifying the magnetic nature of light emission Tremendous advances in the study of magnetic light-matter interactions have recently been achieved using man-made nanostructures that exhibit and exploit an optical magnetic response. However, naturally occurring emitters can also exhibit magnetic resonances in the form of optical-frequency magnetic-dipole transitions. Here we quantify the magnetic nature of light emission using energy- and momentum-resolved spectroscopy, and leverage a pair of spectrally close electric- and magnetic-dipole transitions in trivalent europium to probe vacuum fluctuations in the electric and magnetic fields at the nanometre scale. These results reveal a new tool for nano-optics: an atomic-size quantum emitter that interacts with the magnetic component of light. Magnetic-dipole (MD) transitions at optical frequencies are considered forbidden transitions, because their rates are approximated to be 10 5 times lower than electric-dipole (ED)-allowed transitions [1] . Hence, optics is generally interpreted as a world of electric fields and dipoles. Optical metamaterials exhibiting artificial magnetic response have challenged this notion [2] , [3] , [4] , [5] and helped probe magnetic light-matter interactions [6] , [7] , [8] , [9] . Nevertheless, strong optical-frequency MD transitions do occur in nature. MDs contribute to the intra-4 f electronic transitions of lanthanide ions such as trivalent erbium (Er 3+ ), europium (Eu 3+ ) and terbium (Tb 3+ ) [10] . Today, these rare-earth ions serve as light emitters in a range of technologies from fluorescent lighting to telecom fibre amplifiers, but they have also had an important role in the fundamental study of light-matter interactions. The first MD transition in Eu 3+ was identified as early as 1941 by the elegant technique of wide-angle interference [11] , [12] , and has been revisited within the context of modified spontaneous emission [13] , [14] , [15] , [16] , [17] , [18] . Provided that their emission can be quantitatively distinguished from EDs, MD transitions could serve as active elements for nano-optics. Just as the ED transitions of fluorescent molecules and quantum dots have been used as local sources to control and study electric light-matter interactions [19] , [20] , [21] , [22] , the MD transitions in lanthanides could serve as atomic scale probes of optical magnetic fields [23] , [24] , [25] , [26] , [27] , [28] , and thus help to unravel, enhance and exploit magnetic light-matter interactions at the nanoscale. Here, we directly quantify natural MD transitions in lanthanide ions and leverage them to access the magnetic nature of light emission. To this end, we exploit a method combining optical spectroscopy with Fourier imaging. The resulting energy- and momentum-resolved measurements enable us to decompose luminescence into parts originating from ED and MD transitions, measure their underlying transition dipole moments and use these quantum transitions to independently probe the relative electric and magnetic local density of optical states (LDOS). Distinguishing ED and MD emission ED and MD emission differ in symmetry and polarization. Although both emit into the sine-squared radiation pattern associated with point dipoles, their electric and magnetic field vectors are interchanged. In an inhomogeneous environment, the emission rates and patterns are modified by the interference of directly emitted and scattered fields [13] , [14] , [15] , [16] , [17] , [18] . Differences in these self-interference effects can be exploited to distinguish EDs and MDs based on the different modes into which they emit, even for isotropic emitters like the ions studied here. As an example, Fig. 1a illustrates the different contributions to x -polarized emission into a dielectric substrate ( k x = k y =0) for dipoles embedded within a thin film. Of the three Cartesian dipole orientations that describe an isotropic emitter, only the x -oriented ED and y -oriented MD emit into this mode. The observed emission depends on the interference of the directly emitted light and the wave reflected at the air interface. For normal incidence, the electric field acquires no phase upon reflection at the lower-index air interface. As the phase acquired upon propagation is negligible in this thin film ( D ≪ λ ), the result depends solely on the electric field symmetry of the emitting dipole. For an ED, the electric field is symmetric with respect to the dipole axis, and thus constructive interference will enhance emission into this mode; whereas, the opposite is true for a MD and emission is suppressed. Such interference differences persist for other emission directions and polarizations and in the presence of multiple reflections; in general, the electric and the magnetic LDOS differ in an inhomogeneous environment [29] . Consequently, in a thin film, EDs and MDs can be distinguished by their momentum- and polarization-dependent emission patterns. 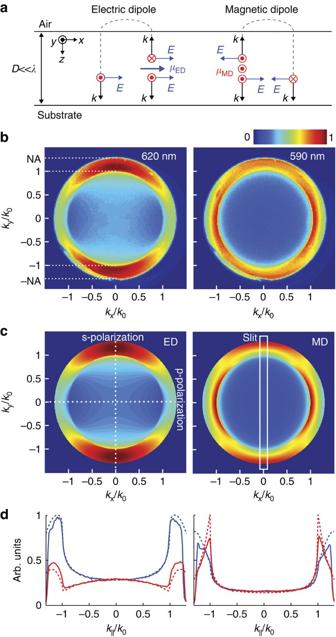Figure 1: Momentum-resolved emission patterns for ED and MD transitions within a thin dielectric film. (a) Schematic illustrating differing self-interference effects for ED and MD emission along thezaxis. The dashed lines indicate the light reflected by the air interface. Owing to opposite field symmetries, ED emission into this mode is enhanced by constructive interference, whereas MD emission is suppressed by destructive interference. (b) Experimental BFP images of Eu3+:Y2O3(D=21 nm,nr=1.77) measured forx-polarized emission with bandpass filters for 605–635 nm and 585–595 nm, respectively. The NA of the objective is 1.3. (c) Theoretical BFP images for a 620-nm isotropic ED emitter and a 590-nm isotropic MD emitter. Dashed lines indicate s- and p-polarized cross-sections, and the solid rectangle shows the region nearkx=0 that is projected onto the entrance slit for energy-momentum spectroscopy. The refractive index of the substrate is taken asnr=1.5. (d) Comparison of the experimental and theoretical cross-sections for s-polarization (blue) and p-polarization (red). Left plot compares experimental data acquired with the 620-nm bandpass filter (solid lines) with the theory for an isotropic ED emitter (dashed lines); right plot compares experimental data acquired with the 590-nm bandpass filter (solid lines) with the theory for an isotropic MD emitter (dashed lines). Figure 1: Momentum-resolved emission patterns for ED and MD transitions within a thin dielectric film. ( a ) Schematic illustrating differing self-interference effects for ED and MD emission along the z axis. The dashed lines indicate the light reflected by the air interface. Owing to opposite field symmetries, ED emission into this mode is enhanced by constructive interference, whereas MD emission is suppressed by destructive interference. ( b ) Experimental BFP images of Eu 3+ :Y 2 O 3 ( D =21 nm, n r =1.77) measured for x -polarized emission with bandpass filters for 605–635 nm and 585–595 nm, respectively. The NA of the objective is 1.3. ( c ) Theoretical BFP images for a 620-nm isotropic ED emitter and a 590-nm isotropic MD emitter. Dashed lines indicate s- and p-polarized cross-sections, and the solid rectangle shows the region near k x =0 that is projected onto the entrance slit for energy-momentum spectroscopy. The refractive index of the substrate is taken as n r =1.5. ( d ) Comparison of the experimental and theoretical cross-sections for s-polarization (blue) and p-polarization (red). Left plot compares experimental data acquired with the 620-nm bandpass filter (solid lines) with the theory for an isotropic ED emitter (dashed lines); right plot compares experimental data acquired with the 590-nm bandpass filter (solid lines) with the theory for an isotropic MD emitter (dashed lines). Full size image To demonstrate this principle, we measured the momentum-distributed luminescence from a Eu 3+ -doped yttrium oxide (Eu 3+ : Y 2 O 3 ) thin film in the Fourier domain by back focal plane (BFP) imaging [30] . Figure 1b shows polarized BFP images obtained using bandpass filters to collect Eu 3+ emission from the 5 D 0 → 7 F 1 and 5 D 0 → 7 F 2 transitions centred at 590 and 620 nm, respectively. These transitions exhibit very different momentum distributions. A comparison with theoretical calculations ( Supplementary Methods ) in Fig. 1c shows that the image for the 620 nm transition resembles an isotropic ED, whereas the image for the 590 nm transition resembles an isotropic MD. The differences are particularly striking for the p-polarized cross-sections (red lines in Fig. 1d ), which are concave down for EDs but concave up for MDs. Such differences allow us to unambiguously differentiate ED and MD emission. Quantifying transitions using energy-momentum spectroscopy As the sample is rotationally symmetric, the s- and p-polarized cross-sections contain all information encoded in the two-dimensional BFP images. Therefore, we can simultaneously characterize the emission in terms of momentum, polarization and wavelength by projecting the BFP image onto the entrance slit of an imaging spectrograph. As illustrated in Fig. 1c , the entrance slit selects emission about k x =0, such that k y = k || . This light is then dispersed by a diffraction grating to obtain an energy spectrum along the x -dimension, and reimaged onto the CCD (charge-coupled device) camera to retain momentum information along the y -dimension. S- or p-polarization states were selected by rotating a polarizer in front of the spectrograph. The resulting BFP spectra, shown in Fig. 2a,b , contain a wealth of information about the emission process. These combined energy-momentum spectra are experimental dispersion diagrams, which show how emission is characteristically distributed into the available optical modes. Integrating over the momentum axis (in the vertical direction) produces an energy spectrum ( Fig. 2c ) of the 5 D 0 → 7 F J transitions in Eu 3+ :Y 2 O 3 (ref. 31 ; see Supplementary Fig. S1 for an energy level diagram of Eu 3+ ). However, by measuring and examining the momentum distribution at different wavelengths ( Fig. 2g ), we can now resolve distinct ED and MD transitions. 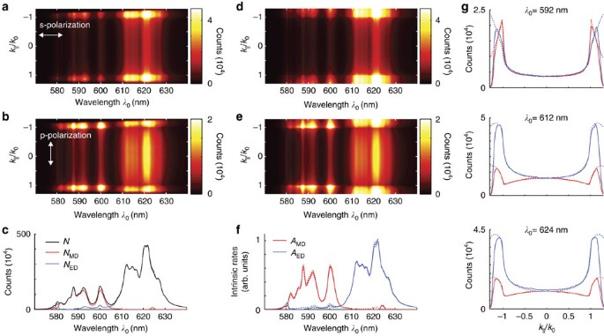Figure 2: Quantifying the ED and MD transitions in Eu3+:Y2O3by energy-momentum spectroscopy. (a,b) Experimental energy- and momentum-resolved BFP spectra for s- and p-polarization, respectively. (c) Integrated energy spectrum showing the total observed emission (N, black line) decomposed into the contributions from ED (NED, blue line) and MD (NMD, red line) transitions. (d,e) Theoretical BFP spectra for s- and p-polarization, respectively, produced using fits to equation (1). (f) Spectrally resolved intrinsic emission rates,AED(solid blue line) andAMD(solid red line), deduced from this fitting analysis together with their 95% confidence intervals (dashed lines). (g) Momentum cross-sections for three representative wavelengths showing strong agreement between experimental data (solid lines) and theoretical fits (dashed lines) for both s-polarization (blue) and p-polarization (red). Emission at 592 nm shows a concave up p-polarized cross-section that is consistent with MD emission, and fitting confirms that this transition is predominantly magnetic (MD=90.8±2.0%). In contrast, 612-nm emission shows a concave down p-polarized cross-section with a local maxima atk||=0, and the fit shows that emission at this wavelength is almost purely electric (ED=99.0±1.0%). Emission at 624 nm shows a less-pronounced maxima, and fitting reveals that this is a more mixed line (ED=88.4±0.7%). Figure 2: Quantifying the ED and MD transitions in Eu 3+ :Y 2 O 3 by energy-momentum spectroscopy. ( a , b ) Experimental energy- and momentum-resolved BFP spectra for s- and p-polarization, respectively. ( c ) Integrated energy spectrum showing the total observed emission ( N , black line) decomposed into the contributions from ED ( N ED , blue line) and MD ( N MD , red line) transitions. ( d , e ) Theoretical BFP spectra for s- and p-polarization, respectively, produced using fits to equation (1). ( f ) Spectrally resolved intrinsic emission rates, A ED (solid blue line) and A MD (solid red line), deduced from this fitting analysis together with their 95% confidence intervals (dashed lines). ( g ) Momentum cross-sections for three representative wavelengths showing strong agreement between experimental data (solid lines) and theoretical fits (dashed lines) for both s-polarization (blue) and p-polarization (red). Emission at 592 nm shows a concave up p-polarized cross-section that is consistent with MD emission, and fitting confirms that this transition is predominantly magnetic (MD=90.8±2.0%). In contrast, 612-nm emission shows a concave down p-polarized cross-section with a local maxima at k || =0, and the fit shows that emission at this wavelength is almost purely electric (ED=99.0±1.0%). Emission at 624 nm shows a less-pronounced maxima, and fitting reveals that this is a more mixed line (ED=88.4±0.7%). Full size image To quantify the nature of emission at each wavelength, we decompose the momentum-distributed emission into parts originating from ED and MD transitions. For this analysis, we make two approximations that have accurately described previous experiments [28] : first, that each ion is an isotropic emitter; second, that the ensemble of ions is effectively homogeneous, that is, the excitation of each emitter results in the same emission spectrum. As all observed emission originates from the same excited level ( 5 D 0 ), we can thus fit the measured counts N s,p ( ω , k || ) to a sum of ED and MD emission (see Supplementary Methods ): where and are the normalized density of optical states into which ED and MD transitions may emit. A ED and A MD are the ED and MD spontaneous emission rates (that is, the spectrally resolved Einstein A coefficients) that would be observed in a homogeneous medium. C is a proportionality constant that depends on sample- and setup-specific experimental parameters, but which only affects the total number of counts and not their energy-momentum distribution. For example, increased non-radiative decay can reduce the total number of observed counts by depleting the single excited level from which all emission originates, but this would not change the radiation pattern or underlying emission rates of ED and MD transitions. In the simplest form, the constant C is given by the product of the time-averaged number of excited ions, the measurement time and a constant related to the spectral calibration of the setup's detection efficiency. Equation (1) highlights how the observed BFP spectra depend on the intrinsic properties of the emitter ( A ED and A MD ) and its local optical environment ( and ). For this known thin-film sample, and can be calculated from analytical expressions ( Supplementary Methods and Supplementary Fig. S2 ). Therefore, fitting experimental data determine the values of A ED and A MD to within the constant C . The fits were performed at each wavelength on the p-polarized data, which contains the most contrast, and over the momentum range of −1.1 k 0 ≤ k || ≤ 1.1 k 0 . (Although the nominal numerical aperture (NA) of the oil immersion objective is 1.3, the effective NA of the experimental setup is lower than this value, and a sharp decrease in the collection efficiency was observed for | k || |>1.1 k 0 .) The resulting energy-momentum spectra ( Fig. 2d,e ) accurately recover the experimental BFP spectra ( Fig. 2a,b ) and momentum curves ( Fig. 2g ) for both polarizations. This procedure decomposes the measured emission spectrum ( Fig. 2c ) into counts originating from ED transitions ( N ED ) and MD transitions ( N MD ). As this decomposition is based exclusively on the momentum dependence of the emission, it is valid even if the ensemble of emitters is not homogeneous (that is, if C was a function of ω ); the origin of the light emitted at each frequency is always encoded in its momentum distribution. The observed percentage of MD counts ( N MD / N ) does, however, depend strongly on the local optical environment and the modes detected (for example, see Supplementary Fig. S3 for measurements highlighting the role of NA on observed MD counts), in addition to the intrinsic properties of the emitter. The intrinsic rates A ED and A MD ( Fig. 2f ) provide a more fundamental and quantitative comparison of competing ED and MD emission processes. These rates are directly related to the transition dipole moments μ ED and μ MD by the following ( Supplementary Methods ): and Even though the contribution of the 5 D 0 → 7 F 1 MD transition appears weaker than the 5 D 0 → 7 F 2 ED transition in Fig. 2c , their intrinsic rates are actually comparable. MD emission is suppressed in this thin-film sample owing to its lowered magnetic density of optical states (as follows from the qualitative argument in Fig. 1a ). We define the intrinsic branching ratios for MD and ED transitions at each frequency: MD( ω )= A MD ( ω )/( A MD ( ω )+ A ED ( ω )) and ED( ω )=1−MD( ω ). For the curves in Fig. 2g , we find that the 592 nm transition is predominantly magnetic (MD=90.8±2.0%) whereas the 612 nm transition is electric (ED=99.0±1.0%). Although Eu 3+ emission is mainly composed of spectrally distinct dipole transitions, the same technique can also be used to quantify degenerate and higher-order transitions. For example, energy-momentum spectroscopy of Tb 3+ :Y 2 O 3 shows that ED and MD contributions can be distinguished even for the strongly mixed 5 D 4 → 7 F 5 Tb 3+ transition ( Supplementary Fig. S4 ). Higher-order transitions, such as electric quadrupoles [32] , also have unique signatures in momentum space [14] , [16] . However, we did not observe evidence for such transitions in the emission spectra of Eu 3+ and Tb 3+ , nor are they expected on the grounds of theory [1] . Using ED and MD transitions to probe the optical environment Having quantified ED and MD emission by energy-momentum spectroscopy, we can use these transitions as local probes of an unknown electromagnetic environment. As a demonstration, we place a several micron thick sheet of mica on top of the Eu 3+ sample with immersion oil ( Fig. 3a ). The measured BFP spectrum ( Fig. 3b ) exhibits rapidly varying interference fringes owing to reflections at the mica–air interface. Of particular interest are the two transitions near 581 nm ( Fig. 3c ). From the analysis in Fig. 2 , these lines have been identified as the 5 D 0 → 7 F 0 ED transition centred at 580.8 nm and the 5 D 0 → 7 F 1 MD transition centred at 582.2 nm. As these lines are spectrally close, their emission probes the same wavelength to a good approximation. Close inspection ( Fig. 3d ) reveals that the momentum-resolved emission patterns for these two transitions are completely inverted. The 180° phase shift observed in these interference fringes is a direct visualization of the symmetry difference between ED and MD emission, as schematically illustrated in Fig. 3a . 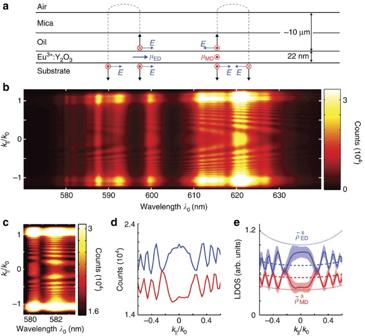Figure 3: Measuring the electric and magnetic local density of states with ED and MD transitions. (a) Schematic illustrating self-interference effects for ED and MD emission near an air–mica interface. The dashed lines indicate the light reflected by the interface. Owing to different field symmetries, the resulting interference is opposite for ED and MD emitters. (b) Experimental s-polarized BFP spectra showing interference fringes characteristic of standing waves formed by the reflection from the interface. (c) Longer-acquisition BFP spectra highlighting the difference between the emissions for the ED transition centred at 580.8 nm and the MD centred at 582.2 nm. (d) S-polarized momentum cross-sections visualizing the symmetry difference between predominantly ED emission at 580.9 nm (blue line) and predominantly MD emission at 581.3 nm (red line). (e) S-polarized relative electric LDOS,(blue), and relative magnetic LDOS,(red). Solid lines show experimental relative LDOS values obtained by fitting the observed counts near 581.1 nm (±0.5 nm), as described in theSupplementary Methods. The shaded regions indicate the 95% confidence intervals for the fits. The dotted and dashed lines show the theoretical LDOS values for two related three-layer systems: air/Eu3+:Y2O3/glass (dotted lines) and oil/Eu3+:Y2O3/glass (dashed lines). To allow for direct comparison, the theoretical results were scaled by a constant factor. Figure 3: Measuring the electric and magnetic local density of states with ED and MD transitions. ( a ) Schematic illustrating self-interference effects for ED and MD emission near an air–mica interface. The dashed lines indicate the light reflected by the interface. Owing to different field symmetries, the resulting interference is opposite for ED and MD emitters. ( b ) Experimental s-polarized BFP spectra showing interference fringes characteristic of standing waves formed by the reflection from the interface. ( c ) Longer-acquisition BFP spectra highlighting the difference between the emissions for the ED transition centred at 580.8 nm and the MD centred at 582.2 nm. ( d ) S-polarized momentum cross-sections visualizing the symmetry difference between predominantly ED emission at 580.9 nm (blue line) and predominantly MD emission at 581.3 nm (red line). ( e ) S-polarized relative electric LDOS, (blue), and relative magnetic LDOS, (red). Solid lines show experimental relative LDOS values obtained by fitting the observed counts near 581.1 nm (±0.5 nm), as described in the Supplementary Methods . The shaded regions indicate the 95% confidence intervals for the fits. The dotted and dashed lines show the theoretical LDOS values for two related three-layer systems: air/Eu 3+ :Y 2 O 3 /glass (dotted lines) and oil/Eu 3+ :Y 2 O 3 /glass (dashed lines). To allow for direct comparison, the theoretical results were scaled by a constant factor. Full size image The fringes in Fig. 3d result from standing waves in the local electric and magnetic fields formed by reflections within the multilayer sample. In any standing wave, the magnetic field maxima correspond to the electric field minima and vice versa, as recently shown at near-infrared wavelengths using nano-structured probes [6] . The quantity measured here, though, is the spontaneous emission from quantum-mechanical transitions between electronic states. Therefore, these measurements probe vacuum fluctuations of the local electric and magnetic fields. Such vacuum fluctuations are directly proportional to the number of optical modes into which an ED or MD may emit and, thus, also proportional to the electric and magnetic LDOS. Using the intrinsic rates A ED and A MD deduced from the bare Eu 3+ :Y 2 O 3 sample and equation (1), we can now extract and , the measured momentum distribution of the relative electric and magnetic LDOS, in this new optical environment (solid lines in Fig. 3e ). These two measured curves oscillate out of phase and about different average values. The rapid oscillations are determined by reflection from the distant mica–air interface, and as discussed above, the maxima of coincide with the minima of . The average values are largely determined by the emitters' immediate optical environment; the measured relative LDOS for the five-layer air/mica/oil/Eu 3+ :Y 2 O 3 /glass sample represents a perturbation on the calculated LDOS for a three-layer oil/Eu 3+ :Y 2 O 3 /glass system (dashed lines in Fig. 3e ). The offset between the measured relative LDOS curves therefore confirms that in the thin, high-refractive index Eu 3+ :Y 2 O 3 film is lower than , as is qualitatively expected from Fig. 1a . Nevertheless, the measured case still shows a significant relative enhancement of as compared with the calculated LDOS for the original sample without oil or mica (dotted lines in Fig. 3e ), because the addition of high-index material near the emitting layer tends to enhance MD transitions. These results highlight the significant role that the optical environment can have on the observed ratio of ED and MD transitions. In conclusion, resolving the natural optical-frequency MD transitions in lanthanide ions provides a new tool for nano-optics: an atomic-size quantum emitter that interacts with the magnetic component of the optical field. As demonstrated here, such MD transitions can be quantified by energy-momentum spectroscopy and used to probe the optical magnetic field and relative LDOS on the nanoscale. The methods presented here are also readily extended to other higher-order transitions, including those recently observed in semiconductor quantum dots [32] . Accessing quantum transitions beyond the ED approximation is of applied as well as fundamental interest. Enhancing and controlling MD emission could have important implications for the many lanthanide-based photonic devices that illuminate our modern world. For example, quantifying the ED and MD transitions in the 1.55 μm line of Er 3+ and characterizing the LDOS in complex waveguide structures could help to improve the design of telecom amplifiers by reducing spontaneous emission noise. The study of higher-order transitions may also have applications in energy-efficient lighting. In fact, the specific ions studied here, Eu 3+ and Tb 3+ , are the common red and green emitters in fluorescent lighting. Despite their names, the forbidden MD transitions of rare-earth ions are neither rare nor forbidden. Sample fabrication We fabricated thin luminescent films of Eu 3+ - and Tb 3+ -doped polycrystalline Y 2 O 3 on quartz coverslips by RF-magnetron co-sputtering in a 90% argon, 10% oxygen gas mixture. Samples were annealed at 1,000 °C for 1 h to activate the emitters. The film thickness was monitored during deposition with a quartz crystal microbalance. Simultaneous deposition on reference silicon substrates enabled the subsequent confirmation of thickness and refractive index via ellipsometry. In the central deposition region from which all luminescent data were acquired, the Eu 3+ :Y 2 O 3 film had a measured thickness ( D ) of 21.6 nm with refractive index ( n r ) of 1.77 to within the accuracy determined from the ellipsometer's repeatability specification. Over the entire deposition region, owing to the configuration of the co-sputtering targets, the maximal observed deviations from these values were D =19 nm, n r =1.82 and D =24.3 nm, n r =1.72. Similarly, in the central deposition region, the Tb 3+ :Y 2 O 3 film had thickness of 14.8 nm with a refractive index of 2.00. Over the entire deposition region, the maximal observed deviations from these values were D =12.4 nm, n r =1.97 and D =16.5 nm, n r =1.95. The effect of sample thickness and refractive index variations on the analysis is discussed in the Supplementary Fig. S5 . 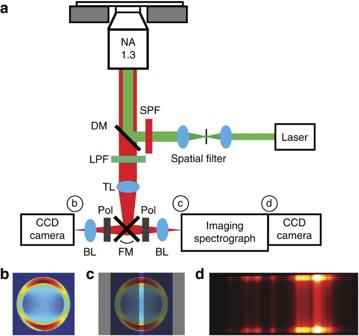Figure 4: Experimental setup used to acquire momentum-resolved BFP images and spectra. (a) Schematic showing the excitation and detection paths for the pump light (green) and collected luminescence (red), respectively. Individual components include the 1.3 NA oil immersion objective, short pass filter (SPF), dichroic mirror (DM), long pass filter (LPF), tube lens (TL), flip mirror (FM), polarizer (Pol) and Bertrand lens (BL). Circled letters indicate the spatial position of the subpanel illustrations: (b) example BFP image recorded directly on a CCD camera, (c) illustration of the BFP image projected onto the entrance slit of the spectrograph and (d) example BFP spectrum recorded on a CCD mounted at the spectrograph exit port. Experimental setup Figure 4 provides a schematic of the experimental setup used to acquire momentum-resolved BFP images and spectra. In both cases, the samples were illuminated in an inverted microscope (Nikon TE2000) through an oil immersion objective (Plan Fluor 100×/1.3 NA) by continuous wave lasers focused to a near diffraction limited spot size (~400 nm). A solid-state 532-nm laser (Coherent Verdi) was used to excite Eu 3+ :Y 2 O 3 , whereas the 488-nm line of an argon ion laser (Coherent Innova) was used to excite Tb 3+ :Y 2 O 3 . For both materials, emission patterns were observed to be independent of excitation polarization, and thus for consistency, all data presented here were acquired with p-polarized linear excitation (that is, with the polarization axis of the excitation source aligned along the slit direction). To acquire two-dimensional momentum images, the BFP of the objective was directly imaged using a Bertrand lens onto a CCD camera (Princeton Instruments Pixis 1024B). To acquire energy- and momentum-resolved spectra, the objective's BFP was imaged onto the entrance slit of an imaging spectrograph (Princeton Instruments SP2300i). After dispersion by a diffraction grating (300 lines mm −1 blazed at 500 nm), the resulting BFP spectra were measured using a CCD camera (Princeton Instruments Pixis 1024B). An intensity-calibrated light source (Princeton Instruments IntensiCal) was used to record the frequency response of the experimental setup, including objective, filters and spectrograph, to within a constant factor. All data are presented and analysed in units of calibrated counts, which have been corrected for the setup's spectral response using 650 nm as a reference point for the constant factor. The integration time used to acquire the experimental data presented in Fig. 1b was 5 s, Fig. 2a,b was 10 s, Fig. 3b was 100 s, Fig. 3c was 600 s and Supplementary Fig. S4a,b was 15 s. Figure 4: Experimental setup used to acquire momentum-resolved BFP images and spectra. ( a ) Schematic showing the excitation and detection paths for the pump light (green) and collected luminescence (red), respectively. Individual components include the 1.3 NA oil immersion objective, short pass filter (SPF), dichroic mirror (DM), long pass filter (LPF), tube lens (TL), flip mirror (FM), polarizer (Pol) and Bertrand lens (BL). Circled letters indicate the spatial position of the subpanel illustrations: ( b ) example BFP image recorded directly on a CCD camera, ( c ) illustration of the BFP image projected onto the entrance slit of the spectrograph and ( d ) example BFP spectrum recorded on a CCD mounted at the spectrograph exit port. Full size image How to cite this article: Taminiau, T.H. et al . Quantifying the magnetic nature of light emission. Nat. Commun. 3:979 doi: 10.1038/ncomms1984 (2012).